Surface changes in the North Atlantic meridional overturning circulation during the last millennium Despite numerous investigations, the dynamical origins of the Medieval Climate Anomaly and the Little Ice Age remain uncertain. A major unresolved issue relating to internal climate dynamics is the mode and tempo of Atlantic meridional overturning circulation variability, and the significance of decadal-to-centennial scale changes in Atlantic meridional overturning circulation strength in regulating the climate of the last millennium. Here we use the time-constrained high-resolution local radiocarbon reservoir age offset derived from an absolutely dated annually resolved shell chronology spanning the past 1,350 years, to reconstruct changes in surface ocean circulation and climate. The water mass tracer data presented here from the North Icelandic shelf, combined with previously published data from the Arctic and subtropical Atlantic, show that surface Atlantic meridional overturning circulation dynamics likely amplified the relatively warm conditions during the Medieval Climate Anomaly and the relatively cool conditions during the Little Ice Age within the North Atlantic sector. Palaeoclimate records from sediments beneath the Florida Current indicate that the Gulf Stream transport decreased by ~10% during the Little Ice Age (LIA) [1] . It has been suggested that decreased meridional heat transport by the Gulf Stream and the North Atlantic Current (NAC) may have been partly responsible for LIA cooling [1] , [2] , [3] , [4] . Instrumental series of Gulf Stream/NAC and Atlantic meridional overturning circulation (AMOC) behaviour and heat transports are limited to a few decades [5] . Given this lack of long instrumental records, information about ocean variability in the North Atlantic on longer timescales can only be obtained from geological proxy archives. To better understand the physical causes of the Medieval Climate Anomaly (MCA) and LIA climate intervals, additional high-quality palaeodata [6] , from diverse geographic settings, including the global oceans, are required to confidently document the spatial and temporal scope of the MCA and LIA. Although the dynamical origins of the MCA and LIA have been widely studied [1] , [3] , [4] , [7] , [8] , [9] , [10] , [11] , [12] , [13] , [14] , [15] , [16] , [17] , [18] , [19] , [20] , [21] , [22] , many aspects of these climate intervals are still poorly characterized and widely debated [4] , [7] , [8] , [9] , [11] , [12] , [13] , [14] , [15] , [16] , [17] , [21] , [22] . Key candidate forcings include external climate drivers (for example, volcanic and solar activity) and internal Earth system feedbacks. Beyond external climate forcings [12] , [20] , it is recognized that natural variability in heat transport via the Gulf Stream and the NAC (which together make up the northward-flowing surface component of the AMOC) to higher latitudes within the Atlantic basin was likely influential in shaping the MCA and LIA climate events [1] , [2] , [3] , [4] . However, this hypothesis has been difficult to test because of a scarcity of suitable precisely dated natural marine proxy archives located within the region of influence of the AMOC. To reconstruct the dynamics of Arctic and Atlantic water masses in this region over the last millennium, we analysed the radiocarbon content of samples obtained from shell growth increments of the long-lived marine bivalve Arctica islandica , which have been absolutely dated using crossdating techniques derived from dendrochronology [23] . The shells used in this study were collected from the North Icelandic shelf at 80 m water depth adjacent to the location of the modern oceanic Polar Front ( Fig. 1 ), a region noted for its sensitivity to surface AMOC changes [24] , [25] , [26] . Because the shell chronology [27] is absolutely dated, 14 C values derived from known-age shell subsamples can be used to precisely constrain the relative 14 C age of water masses. Hence, the absolutely dated radiocarbon data presented here serve as a water mass tracer, rather than as a chronometer. To explore the differences between the global ocean (Marine09) [28] , [29] and the Icelandic shell-derived 14 C record, and to investigate potential causal mechanisms that link the shell 14 C record with North Atlantic Ocean circulation dynamics, we present our radiocarbon data in Δ R format. The Δ R values are determined by the regional deviations in the marine radiocarbon reservoir age from the modelled ocean surface mixed layer reservoir age (Marine09) [28] , [29] , [30] . To first order, Δ R reflects oceanic mixing processes (upwelling, advection) that contribute to the offset between regional and global ocean 14 C ages [30] ; thus, Δ R time series can be used to trace water masses and ocean circulation. North of Iceland, relatively young Atlantic sourced waters (NAC) and relatively old Arctic sourced waters converge and mix ( Fig. 1 ) in the vicinity of the oceanic Polar Front [24] . NAC waters (Δ R values=0 to 50) [24] flow northward and clockwise around West Iceland as the Irminger Current and mix on the North Icelandic shelf with Arctic water (Δ R values >150) [24] , [31] , [32] , flowing southeastward as the East Icelandic Current (a periodic development of the East Greenland Current; Fig. 1 ) [33] . Our findings indicate a declining influence of NAC waters on the North Icelandic shelf during the last millennium. Since circa AD 1940, NAC-derived surface waters have again become more influential north of Iceland and within the Arctic [10] , resembling hydrographic conditions present during the early MCA. We infer that the surface AMOC was relatively strong in Medieval times, became weaker in the LIA, and strengthened again after circa AD 1940. We suggest that the surface component of the AMOC amplified the relatively warm [13] conditions during the MCA and the relatively cool [13] conditions during the LIA within the North Atlantic Ocean. 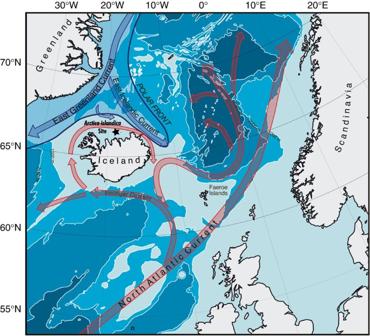Figure 1: Location map of modern ocean surface circulation patterns in the northern North Atlantic. TheA.islandicastudy site on the North Icelandic shelf is shown with a star; map modified from ref.25. Figure 1: Location map of modern ocean surface circulation patterns in the northern North Atlantic. The A . islandica study site on the North Icelandic shelf is shown with a star; map modified from ref. 25 . Full size image Master shell chronology A total of 29 shells (14 dead-collected and 15 live-collected) were used to construct the master shell chronology [27] . The shell chronology [27] extends 1,357 years, and represents the longest continuous annually resolved sclerochronological record ( Fig. 2 ). The mean correlation between all detrended series (Rbar; blue line in Fig. 2c ) [34] is defined only after circa AD 1200, because, before then, sample depth does not exceed two at any point ( Fig. 2e ). The value of Rbar (determined in a 50-year window at 25-year intervals) is low around AD 1200, probably because a prevalence of juvenile specimens in the chronology at that point introduces greater ontogenetic variability. It also falls slightly around AD 1450–1500 and in the late 1700s, indicating a weaker common signal. The Expressed Population Signal (EPS; red line in Fig. 2c ) [35] takes account of both Rbar and the sample depth N (EPS= N ×Rbar/( N ×Rbar+(1−Rbar))) to give an indication of the degree to which the population subsample, included in the chronology, expresses the theoretical population-wide common environmental signal. By convention, EPS ≥0.85 is taken to indicate that the expression of the common signal is adequate [35] . Here the EPS falls below 0.85 only at the start of the period for which it is defined ( circa AD 1200) and during the period AD 1450–1500, when the common signal is relatively weak. It is also notable that EPS does not increase significantly during the twentieth century when the inclusion of a number of live-collected specimens in the chronology raises the sample depth to 15. This indicates that for increment width series that correlate as closely as these, a sample depth between four and six is normally sufficient to provide an adequate signal to noise ratio. The longevity of the animals used here, determined by increment counting and cross-dating, ranks them among the longest lived non-colonial animals known to science. Of particular note are shells 061294 and 061364, which lived for 507 years and 412 years, respectively [27] . These two animals seem to have settled on the sea floor north of Iceland at about the same time ( circa AD 1500), and the raw increment widths from their shells correlate strongly ( r =0.89; P <0.0001) through a period of 410 years ( Fig. 3 ). 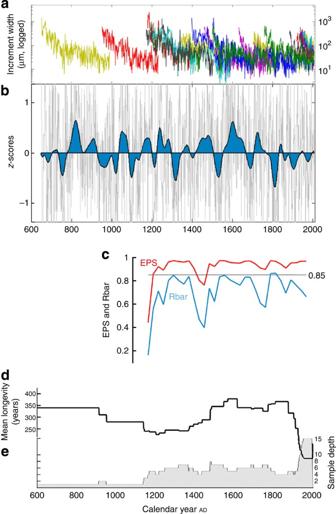Figure 2: Master shell chronology from the North Icelandic shelf and chronology statistics. (a) Raw increment widths (logged) for each of the 29 shells used in the master shell chronology. (b) Detrended growth increments normalized asz-scores ((value−mean)/standard deviation) derived from the autoregressive modelled chronology with a 70-year low pass centrally weighted Gaussian filter; see ref.27for additional details. (c) Expressed population signal (EPS; red) with the 0.85 critical value noted, and the mean correlation between all detrended series (Rbar; blue). (d) Mean longevity of all shells in the chronology at that point. (e) Sample depth of chronology at that point. Figure 2: Master shell chronology from the North Icelandic shelf and chronology statistics. ( a ) Raw increment widths (logged) for each of the 29 shells used in the master shell chronology. ( b ) Detrended growth increments normalized as z -scores ((value−mean)/standard deviation) derived from the autoregressive modelled chronology with a 70-year low pass centrally weighted Gaussian filter; see ref. 27 for additional details. ( c ) Expressed population signal (EPS; red) with the 0.85 critical value noted, and the mean correlation between all detrended series (Rbar; blue). ( d ) Mean longevity of all shells in the chronology at that point. ( e ) Sample depth of chronology at that point. 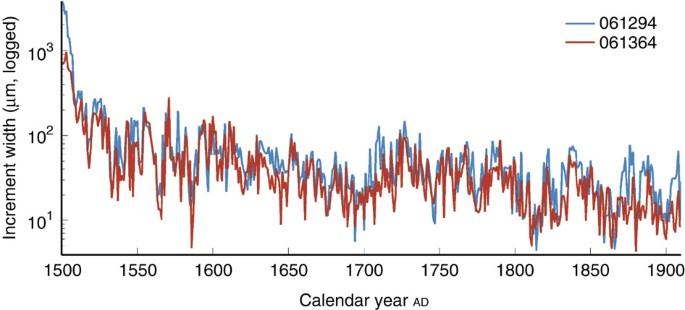Figure 3: Extreme longevity and centuries of synchronous shell growth. Raw increment width measurements (logged here to improve clarity) during a 410-year period (AD1500–1909) for 2 very long-lived specimens ofA.islandica, showing the strength of synchronous growth throughout (r=0.89;P<0.0001;N=410). Full size image Figure 3: Extreme longevity and centuries of synchronous shell growth. Raw increment width measurements (logged here to improve clarity) during a 410-year period ( AD 1500–1909) for 2 very long-lived specimens of A . islandica , showing the strength of synchronous growth throughout ( r =0.89; P <0.0001; N =410). Full size image Origin of radiocarbon signal in shells To determine the likely origin of the radiocarbon signal (atmospheric versus oceanic) in the cross-dated shells, we compared the shell 14 C data with the radiocarbon record for the atmosphere (IntCal09) [28] and the modelled global ocean (Marine09) [28] ( Fig. 4 ). During this interval ( AD 600 to AD 1950), the modelled global ocean [28] , [29] is on average 386 (±39) years older than the atmosphere with respect to radiocarbon ( Fig. 4 ; also see ref. 29 , for a detailed discussion). Further, changes in the global ocean 14 C record are slightly lagged and attenuated compared with the atmosphere. In the early part of the record ( AD 675 to AD 705 and AD 870 to AD 940) (highlighted as Case #1 in Fig. 4 ), the shell-derived 14 C values match the global ocean values. This indicates that a water mass of Atlantic origins (for example, NAC, a water mass that is about 400-years old with respect to radiocarbon) was prevalent on the North Icelandic shelf during the early MCA. Conversely, from AD 1000 to AD 1210, there was a clear departure in shell 14 C values from the global ocean (highlighted as Case #2 in Fig. 4 ) indicating relatively older waters on the North Icelandic shelf; these data are most consistent with a water mass of Arctic origins [24] . This apparent trend (increasing marine radiocarbon reservoir effect) continues into the LIA, until it is briefly interrupted by an atmospheric 14 C pulse from AD 1375 to AD 1400, which is clearly seen in the Marine09 record and the 14 C shell data (highlighted as Case #3 in Fig. 4 ). At least one other atmospheric 14 C perturbation is noted in the shell-based 14 C at ~ AD 1790 (highlighted as Case #4 in Fig. 4 ). During the entirety of the LIA climate interval, waters along the North Icelandic shelf are older than the global ocean. For the first time since the early MCA, shell-based 14 C values equal the global ocean values at AD 1895 and AD 1950, likely indicating a shift to Atlantic-derived waters. Although decadal trends in atmospheric 14 C dynamics are faithfully recorded in the shell record ( Fig. 4 ), the increasing deviation between the Marine09 record and the shell-based radiocarbon signal north of Iceland cannot be explained by atmospheric forcing. 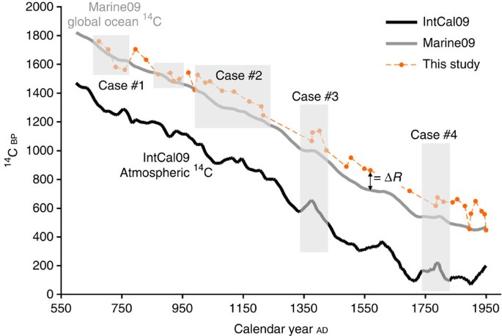Figure 4: Relationship between global and shell radiocarbon datasets. Cross-dated shell-based14C values (this study; solid orange circles) from known-age samples are compared with the atmospheric (IntCal09)28and the global ocean (Marine09)28radiocarbon records fromAD600 toAD1950. In case #1 (early MCA), the shell14C record matches the modelled Marine09 (ref.28) radiocarbon record (marine radiocarbon reservoir effect 386 (±39)28,29). In case #2, the shell14C record deviates from the Marine09 (ref.28) record, indicating a relatively older (with respect to radiocarbon) water mass present on the North Icelandic shelf afterAD950. This long-term deviation between the shell-based and Marine09 radiocarbon records continues into the early twentieth century. Atmospheric14C pulses that are noted in the Marine09 and shell-based radiocarbon records are highlighted as case #3 and #4. An example of ΔR(ref.30) (difference between shell14C age and the Marine0914C age) is noted at ~AD1560 for reference (seeFig. 5).BP=before present (BP=0 atAD1950). Figure 4: Relationship between global and shell radiocarbon datasets. Cross-dated shell-based 14 C values (this study; solid orange circles) from known-age samples are compared with the atmospheric (IntCal09) [28] and the global ocean (Marine09) [28] radiocarbon records from AD 600 to AD 1950. In case #1 (early MCA), the shell 14 C record matches the modelled Marine09 (ref. 28 ) radiocarbon record (marine radiocarbon reservoir effect 386 (±39) [28] , [29] ). In case #2, the shell 14 C record deviates from the Marine09 (ref. 28 ) record, indicating a relatively older (with respect to radiocarbon) water mass present on the North Icelandic shelf after AD 950. This long-term deviation between the shell-based and Marine09 radiocarbon records continues into the early twentieth century. Atmospheric 14 C pulses that are noted in the Marine09 and shell-based radiocarbon records are highlighted as case #3 and #4. An example of Δ R (ref. 30 ) (difference between shell 14 C age and the Marine09 14 C age) is noted at ~ AD 1560 for reference (see Fig. 5 ). BP =before present ( BP =0 at AD 1950). Full size image Changes in Δ R data during the last millennium We present 41 new Δ R shell data (orange circles) spanning AD 675 to AD 1950; the subsamples necessarily integrate several annual increments, so some measurements have a temporal integration of 5 to 20 years ( Fig. 5 ; Supplementary Data 1 ). The Δ R shell values gradually increase over the last millennium, reflecting a shift towards older Arctic-derived water. Decadal- to multi-decadal scale variations in Δ R shell values are most pronounced in the early part of the record and since circa AD 1800. Comparison with known present-day measurements of Δ R (ref. 36 ) indicates that Δ R shell values before and during the early MCA [15] (for example, AD 675-AD 1000) mostly reflect waters derived from an Atlantic (NAC) source, whereas during much of the MCA [15] (after AD 1000) and into the early LIA [24] they indicate a varying mixture of Atlantic and Arctic sources. Progressing into the LIA (after AD 1500), the Δ R shell values are most consistent with a dominant Arctic (East Icelandic Current) source. In AD 1915, the highest Δ R shell value (Δ R =200) is reached. After AD 1915, there is an apparent reversal in Δ R shell values. 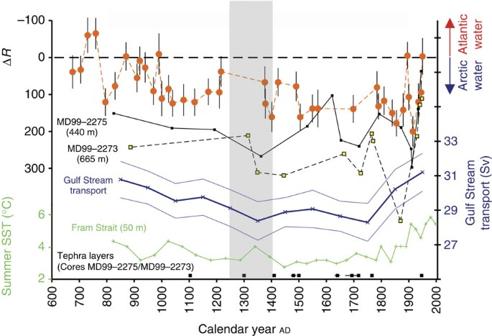Figure 5: Comparison of ΔRdata with other AMOC-sensitive proxy records. Shell-based ΔRvalues (this study; solid orange circles) and sediment-based ΔRvalues24(solid squares; MD99-2275 and MD99-2273) are compared with Gulf Stream transport estimates1(blue) in the Florida Straits and SST values from within the Arctic Ocean10(marine sediment record from Fram Strait off western Svalbard, 79°N; green) during the last millennium. More positive ΔRvalues are representative of Arctic-derived water masses, whereas less positive ΔRvalues are indicative of Atlantic-derived surface waters24. Relatively warmer SST values in Fram Strait indicate a strong Atlantic inflow to the Arctic, while relatively cool SST values likely represent a weak Atlantic inflow to the Arctic10. The errors in the Marine0914C value28and the AMS14C measurement were propagated as random errors yielding a total ΔRshellerror. Tephra layers in marine sediment cores (MD99-2275 and MD99-2273) are shown along the bottom (solid black squares) to illustrate the age control for sediment sequences north of Iceland24. The age/depth models for the Fram Strait and Gulf Stream data are based on linear interpolation between calibrated AMS14C ages, and the Fram Strait data have an age error of about ±30 to 50 years (see ref.10for the full SST record and details); the Gulf Stream data have a possible age error of about ±50 years1. The horizontal grey bar represents the approximate regional timing of the MCA/LIA transition in the marine environment (that is, North Icelandic shelf) noted by refs24,25,26. Figure 5: Comparison of Δ R data with other AMOC-sensitive proxy records. Shell-based Δ R values (this study; solid orange circles) and sediment-based Δ R values [24] (solid squares; MD99-2275 and MD99-2273) are compared with Gulf Stream transport estimates [1] (blue) in the Florida Straits and SST values from within the Arctic Ocean [10] (marine sediment record from Fram Strait off western Svalbard, 79°N; green) during the last millennium. More positive Δ R values are representative of Arctic-derived water masses, whereas less positive Δ R values are indicative of Atlantic-derived surface waters [24] . Relatively warmer SST values in Fram Strait indicate a strong Atlantic inflow to the Arctic, while relatively cool SST values likely represent a weak Atlantic inflow to the Arctic [10] . The errors in the Marine09 14 C value [28] and the AMS 14 C measurement were propagated as random errors yielding a total Δ R shell error. Tephra layers in marine sediment cores (MD99-2275 and MD99-2273) are shown along the bottom (solid black squares) to illustrate the age control for sediment sequences north of Iceland [24] . The age/depth models for the Fram Strait and Gulf Stream data are based on linear interpolation between calibrated AMS 14 C ages, and the Fram Strait data have an age error of about ±30 to 50 years (see ref. 10 for the full SST record and details); the Gulf Stream data have a possible age error of about ±50 years [1] . The horizontal grey bar represents the approximate regional timing of the MCA/LIA transition in the marine environment (that is, North Icelandic shelf) noted by refs 24 , 25 , 26 . Full size image Comparison of Δ R data with other AMOC-sensitive proxy records To establish a more comprehensive reconstruction of Δ R variability along the North Icelandic shelf, we compare our results with sediment-based Δ R values from two high-resolution records [24] (squares) collected from the vicinity of the shell location, but at 440 m (core MD99-2275) and 665 m (core MD99-2273) water depths, respectively ( Fig. 5 ). Because of the positions of these sediment archives, numerous Holocene tephras from Icelandic volcanic sources [37] are available to constrain their age/depth relationship [24] (bottom Fig. 5 ). These records indicate an increase in Δ R values during the last millennium ( Fig. 5 ) consistent with the shell values, but a depth-dependent relationship with Δ R is also apparent. The relationship between water depth and Δ R can be explained by the greater contribution of relatively depleted 14 C water that penetrates onto the shelf at greater depths [24] . All three records show a long-term trend to increasing Δ R values before circa AD 1880, reflecting reduced influence of NAC-derived waters. However, the Δ R data show a large degree of variability after AD 1880, likely indicating increased variability of oceanographic conditions on the North Icelandic shelf. After circa AD 1940, Δ R decreases rapidly towards levels characteristic of the early MCA, suggesting a renewed influence of Atlantic sourced waters on the North Icelandic shelf. Role of upwelling on the Δ R record Although regional upwelling can complicate the interpretation of Δ R , the lack of any covariance ( r 2 =0.01) between co-registered shell carbon isotope (δ 13 C) and 14 C measurements (converted to Δ R values) ( Fig. 6 ; Supplementary Data 1 ), both of which are sensitive proxies of upwelling [38] , strongly indicates that upwelling is not a control on the Icelandic Δ R values. 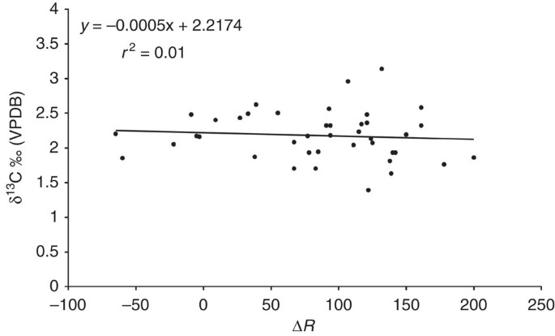Figure 6: Relationship between shell-stable carbon isotope ratios and radiocarbon values. Linear fit and regression statistics for the relationship between co-registered δ13C and14C shell samples (shown here as ΔRvalues). Figure 6: Relationship between shell-stable carbon isotope ratios and radiocarbon values. Linear fit and regression statistics for the relationship between co-registered δ 13 C and 14 C shell samples (shown here as Δ R values). Full size image Even though we are arguing that the long-term trend in Δ R shell values reflects water mass variability, it is possible to make an alternative case that it results from atmospheric 14 C dynamics. By definition, regional Δ R values are derived by subtracting the modelled global ocean 14 C value from the measured 14 C shell value for a given calendar year (in this case, the sclerochronologically determined year) as noted above [30] . The global ocean 14 C value is determined by modelling the atmospheric 14 C record (INTCAL09; see ref. 28 ), which is based on the 14 C content of cross-dated tree-ring records. The model used to assign global ocean 14 C values is based on a simple gas exchange model (for more details see ref. 30 ). As defined by ref. 30 , the Δ R value is composed of two terms: the portion of the shift in regional marine 14 C age attributable to a regional atmospheric 14 C age difference, and an additional shift in marine regional 14 C age, which reflects oceanic processes (such as upwelling and/or advection) that differ from the parameters in the simulated global ocean. Although rapid, decadal-scale atmospheric perturbations in 14 C production seem to impact the Δ R record ( Fig. 4 , Cases #3 and #4), gradual and largely unidirectional changes in 14 C activity in the atmosphere (as noted in INTCAL09 for this interval AD 650 to AD 1950; Fig. 4 ) will not impact the Δ R values, because these changes are also embedded in the Marine09 model, albeit with a slight lag. Because the 14 C Marine09 data are a smoothed version (with appropriate lag times) of the 14 C atmospheric data (for example, INTCAL09), the increasing deviation in Δ R during the last millennium at the study site must be of oceanic origin. Hence, we argue that the Δ R values north of Iceland primarily reflect processes indicative of large-scale ocean circulation dynamics. The proxy transport estimates from the Florida Straits [1] capture a large portion of the northward flow of the Gulf Stream/NAC system ( Fig. 5 ). Comparison of these data with the Δ R values from the North Icelandic shelf suggests that the latter are coupled to Gulf Stream/NAC discharge and the wind-driven (surface) component of AMOC. The associated distinct and converging water masses (Atlantic and Arctic) associated with the oceanic Polar Front ( Fig. 1 ) are largely driven by regional wintertime mean sea-level pressure gradients [39] and wind-stress curl over the region [40] . Hence, changes in regional and basin-scale surface wind patterns, such as the North Atlantic Oscillation (NAO), will in part modulate the flux of Atlantic waters flowing northward to Iceland via the Irminger Current [40] . Over the last millennium, the winter NAO system has been variable, with a strongly positive NAO mode during Medieval times and a neutral to slightly negative NAO mode during the LIA [14] . Over recent decades, the NAO system has been in strong positive mode, similar to the MCA [14] . We hypothesize that the variability in surface AMOC and Δ R values north of Iceland are in part driven by the mean state of the NAO system during the last 1,000 years ( Fig. 7 ). The northerly position of the Gulf Stream wall, Gulf Stream transport, and surface AMOC dynamics are positively correlated with winter NAO values [41] , [42] , [43] , [44] , [45] . Additionally, model results link a strengthened AMOC with a northward shift of the path of the Gulf Stream [45] . Under such conditions, a relatively enhanced transport of Atlantic water is carried northwards as the NAC, ultimately decreasing Δ R values north of Iceland. We infer that the surface component of the AMOC was relatively strong in early Medieval times, became weaker in the LIA, and stronger again after AD ~1940. This inference is corroborated by recent summer sea surface temperature (SST) proxy-based estimates from within the Arctic Ocean [10] (Fram Strait off western Svalbard; 79°N), a region that is also sensitive to surface AMOC dynamics. The Fram Strait SST data [10] indicate that the flux of Atlantic water entering the Arctic Ocean has substantially increased in the last 100 to 200 years ( Fig. 5 ), likely causing a significant portion of the modern Arctic warming [10] . Additionally, the relative strength of Atlantic inflow (and associated heat transport) to Fram Strait was apparently high during the MCA and low during the LIA [10] ( Fig. 5 ). The long-term covariance between Gulf Stream transport estimates and the relative influence of Atlantic and Arctic waters on the North Icelandic shelf ( Fig. 5 ) support the conclusion that the surface strength of the AMOC primarily controls Δ R values north of Iceland. Additionally, sediment-based SST data [24] , [25] , [26] from the North Icelandic shelf and Fram Strait [10] indicate a relatively warm MCA and cold LIA synchronous with the Δ R data and the evolution of Gulf Stream transport. 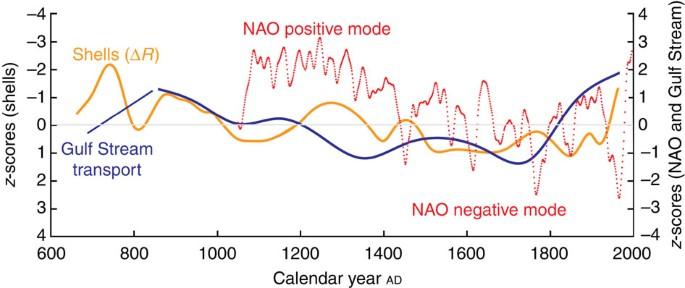Figure 7: Relationship between winter NAO and shell ΔRvalues. z-scores of shell-based ΔRvalues (this study; orange) and Gulf Stream transport estimates (ref.1) (blue) are compared with the raw data used in the wintertime NAO reconstruction (ref.14) (red). Shell ΔRvalues and Gulf Stream transport data were fit with a smoothing spline function (p parameter=0.0003) to highlight the low frequency evolution and coherence of these series. Figure 7: Relationship between winter NAO and shell Δ R values. z -scores of shell-based Δ R values (this study; orange) and Gulf Stream transport estimates (ref. 1 ) (blue) are compared with the raw data used in the wintertime NAO reconstruction (ref. 14 ) (red). Shell Δ R values and Gulf Stream transport data were fit with a smoothing spline function (p parameter=0.0003) to highlight the low frequency evolution and coherence of these series. Full size image Although certain mechanistic and dynamical models link aspects of AMOC behaviour to winter NAO forcing [43] , considerable uncertainty remains regarding the physical mechanisms driving this variability at the decadal- to centennial-scale [46] . The current lack of adequately resolved and well-distributed marine proxy data for the strength of AMOC over the last millennium prevents a rigorous testing of the main factors that modulate surface AMOC variability. Additional work is required to establish the boundary conditions and possible mechanisms (for example, increased volcanism in the thirteenth century [20] and changing Arctic sea ice conditions [47] , [48] ) that led to the inferred surface AMOC weakening and general cooling trend into the LIA climate interval. Despite some progress noted here in documenting the past behaviour of the surface AMOC variability, this study does not reveal any information regarding deepwater formation (rates or volumes) related to AMOC in the northern North Atlantic during this interval. Hence, our understanding of links between the overturning circulation (specifically deepwater formation) and North Atlantic climate, during the last millennium, remains incomplete. The acquisition of high-resolution marine proxy data from regions sensitive to AMOC changes (both surface and deepwater processes) is therefore a major research priority. Shell collection The shells used in this study were part of a collection of live, dead articulated, and dead single valves of A . islandica collected by trawling the seabed surface with a bespoke dredge on the North Icelandic shelf ( Fig. 1 ) in June 2006 from the RV Bjarni Sæmundsson (Cruise No. B05-2006). Shells were collected near the island of Grimsey (66° 31.59′ N, 18° 11.74′ W) at a water depth of 81–83 m (trawl B05AD03) [49] . Radiocarbon analysis To identify shells from long-lived animals that had been alive during the target period and that might therefore be used in an absolutely dated chronology, 24 of the largest and heaviest of the dead-collected shells were initially selected for AMS radiocarbon dating. The periostracum was removed by scraping the outer shell surface using a razor blade near the targeted region and an ~10–30 mg solid sample of shell carbonate was cut and removed from the outer shell surface for radiocarbon sampling. The shell samples were treated following a standard mollusc-rinsing procedure at Aarhus University AMS 14 C Dating Centre (Denmark); to eliminate any possible surface contamination, the outer 25% of the shell was removed by etching in 1 M HCl. Any organic carbon incorporated in the shell carbonate was removed by treatment with a KMnO 4 solution for 16–20 h at 80 °C. The CO 2 was liberated with ~100% phosphoric acid in an evacuated vial at 25 °C. Part of the CO 2 was used for δ 13 C measurements; the remainder was converted to graphite for AMS 14 C measurements on the Centre's EN tandem accelerator by reduction with H 2 , with cobalt as a catalyst. Shell chronology Additional detailed methods regarding the construction of the master shell chronology are outlined in ref. 27 . In brief, the shell valves were sectioned along the axis of maximum growth from the hinge tooth at the umbo to the outer shell margin. The exposed surface was ground and polished, then etched in one of two ways: either in a modified Mutvei solution [49] , [50] or in 0.1 M HCl for 2 to 4 min (ref. 51 ). An acetate peel replica was taken of the etched surface from which the annual growth increments could be viewed under transmitted light and measured using dedicated software (see ref. 49 for additional details). Of the 24 dead-collected shells that were radiocarbon dated, 6 were dated before the target period and a further 4 could not be reliably measured because their increments could not be visualized with sufficient resolution. The other 14 were measured and cross-dated and, in all cases, their sclerochronologically determined calendar ages were found to be consistent with their calibrated radiocarbon ages. Growth in A . islandica is similar to growth in trees in that it is characterized by strong ontogenetic trends in increment width and variance [23] . These trends can be removed with the same detrending techniques that are used in dendrochronology. For crossdating, the measured growth increment series were high-bandpass-filtered by taking residuals from a 15-year spline applied to the logarithms of the increment widths [51] . For chronology construction, lower frequency variability was preserved by taking residuals from a negative exponential function applied to a data adaptive power transformation of the raw increment width series [52] . The dendrochronology software ARSTAN was used to construct the chronology as an autoregressively modelled biweight robust mean function of the detrended increment width series (ARSTAN for WINDOWS 41d; ref. 53 ). Sample depth is at least 4 after AD 1194. The shell record has been extended to AD 649 with the addition of two index series (shell 061312 and shell 061664). Shell 061312 correlates significantly with the chronology (mean value of 4 series excluding 061312), during AD 1200–31 ( r =0.69; N =32; P <0.001), and shell 061664 correlates significantly with 061312 during AD 952-88 ( r =0.61; N =37; P <0.001). Pending the identification of coeval shells that can be used to increase the sample depth and strengthen the dating model during this period, absolute dating earlier than AD 1194 cannot be guaranteed. The master shell chronology is cross-dated (minimum replication of 4 shells) from AD 1194 to AD 2005. The mean longevity of the shells in the chronology generally exceeds 200 years ( Fig. 2d ), dropping only after AD 1934 when several live-collected shells enter the chronology. Eight of the shells used in the chronology are from animals, which lived for more than 300 years. Calculation of Δ R To determine the deviation in the local marine radiocarbon reservoir age (Δ R ) north of Iceland, the modelled ocean (via Marine09; see ref. 28 ) 14 C value, for the sclerochronologically determined calendar year of the sample, was subtracted from the 14 C shell value determined by AMS dating (see ref. 30 and Supplementary Data 1 ). Updated Δ R values for shells 061294 and 061315 The individual specimen (shell 061294) reported here as having lived for 507 years has previously been reported with a lifetime of 405-to-410 years [49] . This adjustment was a consequence of a refinement in the method of increment counting [27] . Previously, when working with shells from UK waters with lifetimes of up to 250 years, measurement in the hinge-plate region was recommended [51] , because the increments there were less vulnerable to the disturbance caused by external shocks and were generally easier to visualize. A. islandica from the North Icelandic shelf, however, are more long-lived than those from UK waters [23] , [27] , [51] and are also slightly smaller. In these shells, the smaller increments in the hinge plate can be so tightly packed that they can no longer be distinguished, and it is possible for groups of narrow increments to be counted as a single increment. Subsequent to the initial report of the longevity of shell 061294, it was remeasured on the outer shell margin and cross-dated ( Fig. 3 ) with other contemporary specimens, thus confirming the redetermined longevity, highlighting the utility of crossdating and emphasizing the high level of synchronous growth in A. islandica populations. The Δ R values reported here for shells 061294 and 061315 reflect the adjustments of the sclerochronological years of the samples taken for radiocarbon analysis, and the Δ R values for shells 061294 and 061315, reported by ref. 49 , are superseded by values reported here ( Supplementary Data 1 ). Statistical evaluation of the millennial-scale Δ R shell trend To test whether the Δ R shell trend is statistically significant before the modern Δ R shell transition ( Fig. 5 ), we fit the data ( AD 675 to AD 1915) with a simple linear regression model ( Fig. 8 ). On the basis of the regression statistics ( r 2 =0.35; P <0.0001) and the fact that the model results (95% confidence interval; Curve Fitting Toolbox in MatLab R2010A) do not overlap (shown by the highlighted rectangles) in the early and late parts of the record, we conclude that the Δ R shell trend during the last millennium is robust and statistically valid. We only modelled data from AD 675 to AD 1915, because the most positive Δ R values in the shells and sediments occurred around AD 1915. 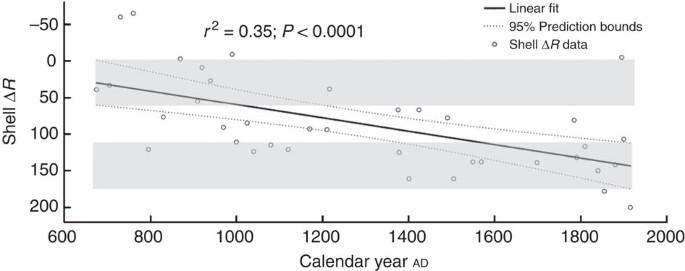Figure 8: Millennial-scale trend in shell ΔRvalues. Linear fit and regression statistics of the shell ΔRdata (AD675 toAD1915) are shown. The data were modelled (solid black line) using MatLab (version R2010A; Curve Fitting Toolbox) to establish the uncertainty in modelled shell ΔRdata. The 95% (confidence interval) prediction bounds (dashed lines) of the model are shown, and these results illustrate that the prediction bounds do not overlap between the early and late parts of the record (highlighted rectangles). Figure 8: Millennial-scale trend in shell Δ R values. Linear fit and regression statistics of the shell Δ R data ( AD 675 to AD 1915) are shown. The data were modelled (solid black line) using MatLab (version R2010A; Curve Fitting Toolbox) to establish the uncertainty in modelled shell Δ R data. The 95% (confidence interval) prediction bounds (dashed lines) of the model are shown, and these results illustrate that the prediction bounds do not overlap between the early and late parts of the record (highlighted rectangles). Full size image How to cite this article: Wanamaker, A. D. et al . Surface changes in the North Atlantic meridional overturning circulation during the last millennium. Nat. Commun. 3:899 doi: 10.1038/ncomms1901 (2012).